Tuning the magneto-structural properties of non-porous coordination polymers by HCl chemisorption Responsive materials for which physical or chemical properties can be tuned by applying an external stimulus are attracting considerable interest in view of their potential applications as chemical switches or molecular sensors. A potential source of such materials is metal-organic frameworks. These porous coordination polymers permit the physisorption of guest molecules that can provoke subtle changes in their porous structure, thus affecting their physical properties. Here we show that the chemisorption of gaseous HCl molecules by a non-porous one-dimensional coordination polymer instigates drastic modifications in the magnetic properties of the material. These changes result from profound structural changes, involving cleavage and formation of covalent bonds, but with no disruption of crystallinity. The design of responsive magnetic materials is one of the hot topics in molecular magnetism. In this area, coordination chemistry is having a key role by providing remarkable examples of molecule-based materials in which magnetic properties can be reversibly tuned at low temperatures through a physical stimulus, such as light [1] , [2] or pressure [3] , [4] . With the recent explosion in research on metal organic frameworks (MOFs) [5] , [6] , [7] , [8] , [9] , [10] , the use of a chemical stimulus such as gas sorption to affect the magnetic properties of a porous coordination polymer has also been explored [11] . However, the synthesis of magnetic MOFs is a challenging issue, as long-range magnetic ordering and porosity are inimical to one another: magnetic cooperativity due to exchange interactions is favoured with short distances, whereas porosity is enhanced with long linkers [12] . A possible approach to overcome this challenge consists of taking advantage of the sensitivity of spin-crossover complexes to subtle structural changes in metal coordination environments, which do not require magnetic cooperativity [13] , [14] , [15] . Thus, it has been shown that MOFs based on these molecular complexes exhibit magnetic switching at room temperature on physisorption of specific molecules within the porous framework [16] , [17] . The high sensitivity of these materials is also evidenced by the modification of the transition temperature on oxidative addition reactions following gas sorption at metal sites that are far from the magnetic centres [18] , [19] . A different approach to tune the magnetic properties of porous solids consists of the modification of the magnetic ground state of the MOF, which can be achieved through gas sorption processes that subtly affect the geometry of either the bridge between metal centres [20] or the ligand substituents [21] . The change of the oxidation state of the metal centre [22] or the variation of the coordination number [23] on hydration/dehydration has also been used to modify the magnetic properties of porous materials. In all these cases, the presence of pores is essential to accommodate the gas molecules that induce the minor structural changes in the framework provoking major changes in the magnetic properties. However, it has been shown that changes in the metal coordination environment might also be feasible in non-porous materials through the chemisorption of some molecular species [24] . A particular example of such a dramatic transformation involves the reaction of molecular solids with gaseous HX (X=Cl, Br) leading to profound structural changes [25] , [26] , where porosity is not necessary, as the chemisorption process involves the removal/addition of HX from/to the framework itself. The observation that non-porous molecular crystals are able to sorb HX prompted us to explore whether this chemisorption process could be used as an approach to design responsive molecular materials with tunable magnetic properties, which would permit the uptake of gases in the absence of pores to alleviate the difficulty in combining porosity and magnetic cooperativity. Here we show that on chemisorption of three equivalents of HCl molecules, the crystalline coordination compound [Cu(pyim)(Cl)(MeOH)] [ 1 , where pyimH=2-(imidazol-2-yl)pyridine] changes its structure from a polymeric chain of pentacoordinated square-pyramidal Cu centres to an ionic solid, (H 2 pyimH)[CuCl 4 ] ( 2 ), containing discrete distorted tetrahedral [CuCl 4 ] 2− anions. Compound 2 is able to extrude two equivalents of HCl yielding the molecular compound cis -[CuCl 2 (pyimH)] ( 3 ) in which the Cu centres present a square-planar geometry. The remarkable concerted rearrangement of covalent bonds that occurs during the sorption/desorption processes results in dramatic changes in the magnetic properties of the materials, from strong antiferromagnetic interactions in 1 to weak ferro- or antiferromagnetic interactions in 2 and 3 , respectively. This can be precisely understood because of the retention of crystallinity of the materials. The single-crystal nature of compounds 1 and 2 provides direct structural evidence of the profound structural changes as a result of the sorption process, whereas complete structure determination for compound 3 was carried out by ab initio synchrotron X-ray powder diffraction (XRPD) analysis, as the removal of the gas molecules yields a uniform microcrystalline powder. Synthesis and structure of non-porous coordination polymer 1 The controlled reaction of CuCl 2 ·2H 2 O and pyimH under basic conditions results in green needle-shaped crystals of 1 after several weeks. Structural analysis by X-ray single-crystal diffraction at 120 K revealed that 1 is composed of helical one-dimensional chains that run parallel to the crystallographic c -axis ( Fig. 1 ). Individual crystals are chiral, but single crystals of both chiralities (space groups P 3 2 and P 3 1 ) are found in the product ( Fig. 2 ), which is a racemic mixture. Fully deprotonated [pyim] − ligands connect adjacent Cu centres via the imidazolate moieties within the ligands, forming a Cu–NCN–Cu bridge, which is reminiscent of that found in the recently discovered zeolitic imidazolate frameworks [27] , [28] and that has been exploited to promote magnetic interactions in Cu II dimers [29] . The ligand pyimH has been previously used in the synthesis of mononuclear spin-crossover complexes acting as a bidentate ligand [30] , but its deprotonation to act as a tridentate ligand for the formation of a coordination polymer is unprecedented. The Cu–N distances are 1.969(7), 1.979(7) and 2.034(7) Å. The coordination sphere of the metal centres is completed with terminal Cl and MeOH ligands [Cu–Cl: 2.274(2), Cu–O: 2.277(7) Å], resulting in a distorted square pyramidal pentacoordinated Cu centre. Each helical chain interacts with six neighbouring independent chains via O–H···Cl hydrogen bonds [31] between the methanol and chloride ligands ( Fig. 2 ). 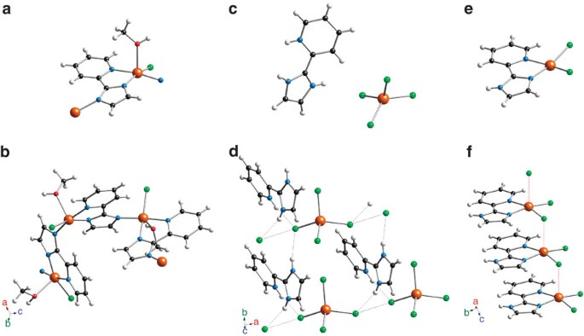Figure 1: Crystal structures of 1, 2 and 3. (a) Structural unit of1showing the distorted square pyramidal pentacoordinated Cu centre and the bridging [pyim]−ligand. (b) View of the helical one-dimensional coordination polymer1, which runs parallel to the crystallographicc-axis. The Cu–NCN–Cu bridge provides the closest contacts between the Cu centres. (c) Structural unit of salt2showing the distorted tetrahedral [CuCl4]2−anions and [H2pyimH]2+cations. (d) Crystal structure of2showing the two-dimensional hydrogen-bonded network formed by N–H···Cl–Cu hydrogen bonds. Each cation interacts with three anions via two N–H···Cl–Cu and one asymmetrically bifurcated N–H···Cl2Cu hydrogen bonds, whereas intermolecular Cu–Cl···Cl–Cu interactions provide the closest contacts between [CuCl4]2−anions. (e) Structural unit of3in which the Cu centres adopt acissquare-planar geometry and the chelating ligand [pyimH] remains neutral. (f) One-dimensional coordination network structure of3formed through a weak apical interaction with one of the chlorine atoms of a neighbouring complex. Cu–Cl···Cu interactions are the closest contacts between the Cu centres. Key: Cu, orange; Cl, green; N, blue; O, red; C, black; H, white. Dotted lines represent non-covalent interactions. Figure 1: Crystal structures of 1, 2 and 3. ( a ) Structural unit of 1 showing the distorted square pyramidal pentacoordinated Cu centre and the bridging [pyim] − ligand. ( b ) View of the helical one-dimensional coordination polymer 1 , which runs parallel to the crystallographic c -axis. The Cu–NCN–Cu bridge provides the closest contacts between the Cu centres. ( c ) Structural unit of salt 2 showing the distorted tetrahedral [CuCl 4 ] 2− anions and [H 2 pyimH] 2+ cations. ( d ) Crystal structure of 2 showing the two-dimensional hydrogen-bonded network formed by N–H···Cl–Cu hydrogen bonds. Each cation interacts with three anions via two N–H···Cl–Cu and one asymmetrically bifurcated N–H···Cl 2 Cu hydrogen bonds, whereas intermolecular Cu–Cl···Cl–Cu interactions provide the closest contacts between [CuCl 4 ] 2− anions. ( e ) Structural unit of 3 in which the Cu centres adopt a cis square-planar geometry and the chelating ligand [pyimH] remains neutral. ( f ) One-dimensional coordination network structure of 3 formed through a weak apical interaction with one of the chlorine atoms of a neighbouring complex. Cu–Cl···Cu interactions are the closest contacts between the Cu centres. Key: Cu, orange; Cl, green; N, blue; O, red; C, black; H, white. Dotted lines represent non-covalent interactions. 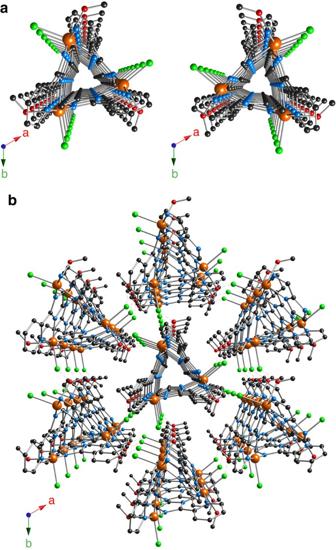Figure 2: Structural view of coordination polymer 1. (a) Helical one-dimensional chains of compounds1+(left, space groupP32), and1–(right, space groupP31) viewed along thecaxis. Individual crystals are chiral but the product is a racemic mixture where single crystals of both chiralities are found. (b) Crystal structure of compound1+showing the interaction of one chain with six neighbouring independent chains via O–H···Cl hydrogen bonds (dashed red lines) between the methanol and chloride ligands. Hydrogen atoms have been omitted for clarity. Key: Cu, orange; Cl, green; N, blue; O, red; C, black; H, white. Full size image Figure 2: Structural view of coordination polymer 1. ( a ) Helical one-dimensional chains of compounds 1+ (left, space group P 3 2 ), and 1– (right, space group P 3 1 ) viewed along the c axis. Individual crystals are chiral but the product is a racemic mixture where single crystals of both chiralities are found. ( b ) Crystal structure of compound 1+ showing the interaction of one chain with six neighbouring independent chains via O–H···Cl hydrogen bonds (dashed red lines) between the methanol and chloride ligands. Hydrogen atoms have been omitted for clarity. Key: Cu, orange; Cl, green; N, blue; O, red; C, black; H, white. Full size image Chemisorption/desorption of gaseous HCl molecules Coordination polymer 1 is stable under ambient conditions, but possesses reactive Cu centres that undergo ligand substitution when a crystalline sample is exposed to an atmosphere of hydrochloric acid vapour in a sealed vessel, despite the lack of pores in the structure ( Fig. 2 ). Thus, this process requires the cooperative movement of atoms in the solid state. Despite the retention of crystallinity, the sorption process causes breaks in the single crystals and, predominantly, yields a polycrystalline powder. However, we were able to isolate one single crystal after the HCl chemisorption that permitted the structural analysis of the product (H 2 pyimH)[CuCl 4 ], 2 . The sorption process leads to protonation of the imidazolate ligand and modifies the geometry around the Cu centres, as indicated by a dramatic colour change from dark green to yellow within a few minutes. The chemisorption of HCl occurs in 100% yield within 1 h, as demonstrated unequivocally by XRPD and electron paramagnetic resonance (EPR) spectroscopy ( Supplementary Figs S1 and S2 ). Three equivalents of HCl molecules are inserted into all Cu–N bonds requiring rupture of the covalent bond of the gaseous molecules (H–Cl) and of the coordination bonds of the polymeric compound so that new N–H and Cu–Cl bonds can be formed. In addition, the MeOH molecules that complete the coordination sphere in 1 are displaced during the sorption process. The resultant hydrogen-bonded salt comprises distorted tetrahedral [CuCl 4 ] 2− anions and (H 2 pyimH) 2+ cations that form a 2D network of (6,3) topology in which each cation interacts with three anions via two N–H···Cl–Cu hydrogen bonds (H···Cl 2.162 and 2.184 Å) and one asymmetrically bifurcated N–H···Cl 2 Cu hydrogen bond (H···Cl 2.383 and 2.798 Å) ( Fig. 1 ). Intermolecular Cu–Cl···Cl–Cu interactions [3.631(2) Å] provide the closest contacts between [CuCl 4 ] 2− anions, which form supramolecular chains along the a -axis. When left to stand in air at room temperature, 2 is able to release two equivalents of HCl gas leading to conversion into cis -[CuCl 2 (pyimH)], 3 . The HCl molecules that are liberated are part of the components of the framework, which implies that porosity is not needed for the release reaction to take place. Rather, a complete rearrangement of the solid takes place ( Fig. 3 ). Interestingly, only the least acidic of the three N–H groups (pK a =13.4(1) in water) [32] , which also forms the longest N–H···Cl hydrogen bond, does not participate in the dehydrochlorination process. This clearly confirms the significant role of the N–H···Cl hydrogen bonds in this type of reaction [33] . The complete deprotonation of the ligand pyimH requires the use of basic conditions. The resultant compound from the extrusion of two equivalents of HCl molecules is a green polycrystalline powder whose structure has been determined ab initio by XRPD and refined by Rietveld analysis ( Fig. 4 ), as all attempts to recrystallize it from solution yielded a microcrystalline powder. The structure of 3 consists of neutral [CuCl 2 (pyimH)] units in which the copper atoms adopt a cis square-planar geometry coordinated by two nitrogen atoms from pyimH and two chloride ligands ( Fig. 1 ) [Cu–N distances: 1.951(5) and 2.117(5) Å; Cu–Cl distances: 2.195(5) and 2.255(5) Å]. A one-dimensional coordination network structure is formed through a weak apical interaction with one of the chlorine atoms of a neighbouring complex [Cu–Cl···Cu 2.846(5) Å]. These chains are linked into 2D layers through N–H···Cl hydrogen bonds involving the imidazole group and chloride ligand and weaker C–H···Cl hydrogen bonds provide intermolecular links in the third dimension. This hydrogen bond donor capacity of chelated pyimH has been previously reported in mononuclear Fe II spin-crossover systems [34] . Remarkably, when subjected to an atmosphere of HCl vapour, compound 3 is able to incorporate two equivalents of this gas and the resulting crystalline product was confirmed to be salt 2 , showing that the molecular coordination compound 3 and the salt 2 can be interconverted as crystalline solids at room temperature. The sorption behaviour of compound 3 is therefore analogous to that of compound 1 with the proviso that only two equivalents of HCl are incorporated. Thus, compound 3 can be seen as a likely intermediate in the uptake of three equivalents of HCl by 1 to yield 2 via a two-step process: an irreversible sorption of one equivalent of HCl ( 1 → 3 ) followed by a reversible sorption of two equivalents of HCl ( 3 2 ). On exposure of 1 to HCl vapours in the magnetic sample holder, the material closer to the vapours of HCl began to change colour from dark green to light green ( Supplementary Fig. S3 ). This colour front moved along the capillary over time providing a visual indication of the reaction front, which is completed in less than 1 h. On further exposure, a second colour front (light green-to-yellow) is observed, and indicates completion in 1 day. This strongly suggests that the chemisorption process 1 → 2 is a two-step process that occurs via the formation of 3 . Interestingly, all attempts to prepare crystalline 2 from aqueous solution by reaction of CuCl 2 with one equivalent of pyimH in concentrated HCl afforded only a microcrystalline powder of 3 . Thus, the synthesis of 2 is only achievable by a gas-solid reaction with either 1 or 3 as the starting material. We speculate that this is due to the process being a gas–solid equilibrium reaction analogous to previous studies [35] , but the chelating effect of the ligand pyimH affects the position of the equilibrium. 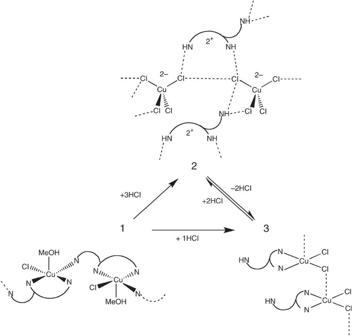Figure 3: Rearrangement of covalent bonds on chemisorption and release of HCl. When crystalline [Cu(pyim)(Cl)(MeOH)]1is exposed to an atmosphere of hydrochloric acid vapour an irreversible sorption of 3 equivalents of HCl (1→2) results into the hydrogen bonded salt (H2pyimH)[CuCl4],2, which is able to release two equivalents of HCl gas in a complete rearrangement of the solid, leading to conversion intocis-[CuCl2(pyimH)],3, which is capable of reversibly incorporate two equivalents of HCl affording2(23). Alternatively,3can also be obtained by direct exposition of1to one equivalent of HCl (1→3). Chemisorption of HCl molecules involves insertion into Cu–N bonds requiring rupture and formation of new covalent bonds. Figure 3: Rearrangement of covalent bonds on chemisorption and release of HCl. When crystalline [Cu(pyim)(Cl)(MeOH)] 1 is exposed to an atmosphere of hydrochloric acid vapour an irreversible sorption of 3 equivalents of HCl ( 1 → 2 ) results into the hydrogen bonded salt (H 2 pyimH)[CuCl 4 ], 2 , which is able to release two equivalents of HCl gas in a complete rearrangement of the solid, leading to conversion into cis -[CuCl 2 (pyimH)], 3 , which is capable of reversibly incorporate two equivalents of HCl affording 2 ( 2 3 ). Alternatively, 3 can also be obtained by direct exposition of 1 to one equivalent of HCl ( 1 → 3 ). Chemisorption of HCl molecules involves insertion into Cu–N bonds requiring rupture and formation of new covalent bonds. 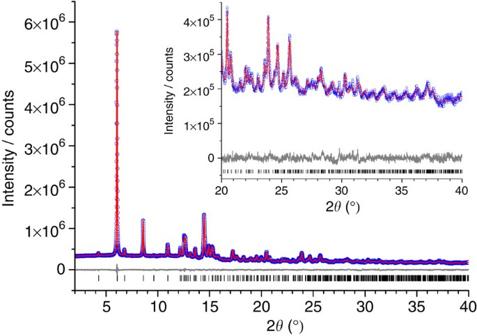Figure 4: X-ray powder pattern and Rietveld refinement of compound3. Observed (blue) and calculated (red) powder XRPD pattern profiles and difference plot [(Iobs−Icalcd)] (grey) of the Rietveld refinement of a polycrystalline sample of3collected at room temperature in the 2θrange 2.0–40.0° using λ=0.826134 Å. Rietveld refinement afterab initiostructure solution converged toRwp=0.02267,R′wp=0.07678 (R′wpis the background-subtractedRwp). The inset shows an expansion of the high angle region. Full size image Figure 4: X-ray powder pattern and Rietveld refinement of compound 3 . Observed (blue) and calculated (red) powder XRPD pattern profiles and difference plot [( I obs − I calcd )] (grey) of the Rietveld refinement of a polycrystalline sample of 3 collected at room temperature in the 2 θ range 2.0–40.0° using λ=0.826134 Å. Rietveld refinement after ab initio structure solution converged to R wp =0.02267, R ′ wp =0.07678 ( R ′ wp is the background-subtracted R wp ). The inset shows an expansion of the high angle region. Full size image Magnetic response to HCl chemisorption Major changes in the magnetic properties take place on HCl chemisorption/desorption as a consequence of the structural changes experienced by the compounds, which modify the magnetic exchange paths between the copper centres as well as the coordination sites ( Fig. 5 ). The magnetic characterization of compound 1 shows that the product of the molar magnetic susceptibility and temperature, χ M T , has a value of 0.38 emu K mol −1 at room temperature ( Fig. 5 ). As the system is cooled, the χ M T product decreases continuously, indicating the presence of strong antiferromagnetic Cu–Cu interactions through the imidazolate bridges. The magnetic data have been analysed using a model for a linear antiferromagnetic chain of spin=½. This fit leads to a magnetic coupling J =−65.4 cm −1 ( Supplementary Fig. S4 ), using a Landé-factor g =2.13 as measured by EPR ( Supplementary Fig. S2 ). A small fraction of the paramagnetic monomer is also detected at low temperatures (contribution of ca. 8%). 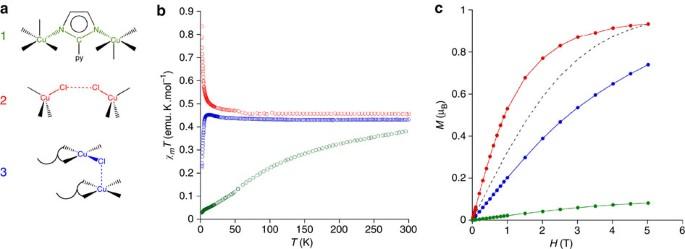Figure 5: Magnetic response to HCl chemisorption. (a) Different magnetic superexchange paths for each compound: the Cu–NCN–Cu imidazolate bridge in1is shown in green; the two-halide Cu–Cl···Cl–Cu exchange pathway in2is shown in red; the Cu–Cl···Cu chloride bridge in3is shown in blue. (b) Thermal dependence of theχMTproduct of1(green),2(red) and3(blue) in the temperature range 2–300 K after the solid–gas reactions indicating the presence of strong antiferromagnetic Cu–Cu interactions in1, weak ferromagnetic interactions in2and weak ferromagnetic interactions coexisting with a dominant antiferromagnetic coupling in3. (c) Field dependence of the magnetization,M, measured at 2 K of compounds1(green),2(red) and3(blue) and the Brillouin function for (black dashed line), which confirms the magnetic features of1–3. Figure 5: Magnetic response to HCl chemisorption. ( a ) Different magnetic superexchange paths for each compound: the Cu–NCN–Cu imidazolate bridge in 1 is shown in green; the two-halide Cu–Cl···Cl–Cu exchange pathway in 2 is shown in red; the Cu–Cl···Cu chloride bridge in 3 is shown in blue. ( b ) Thermal dependence of the χ M T product of 1 (green), 2 (red) and 3 (blue) in the temperature range 2–300 K after the solid–gas reactions indicating the presence of strong antiferromagnetic Cu–Cu interactions in 1 , weak ferromagnetic interactions in 2 and weak ferromagnetic interactions coexisting with a dominant antiferromagnetic coupling in 3 . ( c ) Field dependence of the magnetization, M , measured at 2 K of compounds 1 (green), 2 (red) and 3 (blue) and the Brillouin function for (black dashed line), which confirms the magnetic features of 1 – 3 . Full size image HCl chemisorption results in the protonation of the [pyim] − ligand, which switches off the efficient Cu–Cu exchange pathway present in 1 , and therefore the Cu II spins do not show any interaction down to 20 K in compound 2 , as demonstrated by the constant χ M T value of 0.45 emu K mol −1 observed from 300 to 20 K. On further cooling, χ M T increases to reach a value of 0.83 emu K mol −1 at 2.0 K ( Fig. 5 ), indicating the presence of a weak ferromagnetic exchange coupling of J =+0.75 cm −1 ( Supplementary Fig. S4 ). The most plausible exchange pathway in 2 involves a two-halide Cu–Cl···Cl–Cu interaction ( Fig. 5a ) [36] , [37] , although it may also contain some influence from other potential superexchange mechanisms, such as Cu–Cl···Cu interactions or N–H···Cl–Cu hydrogen bonds. Because of the rapid release of HCl by 2 (conversion to 3 ), magnetic measurements were performed under HCl atmosphere to guarantee homogeneity during the magnetic measurements. After release of HCl, the magnetic behaviour of 3 indicates that the Cu–Cu interactions are also very weak ( Fig. 5 ), which is due to the fact that after the release of two equivalents of HCl ( 2→3 ) the imidazole ligand remains neutral and does not act as a bridging ligand in the product. Instead, a chloride ligand bridges the square-planar Cu II units. Similar to 2 , exchange interactions are only detected in the low-temperature magnetic behaviour. Below 20 K χ M T increases slightly to reach a maximum value of 0.45 emu K mol −1 at 13 K and then decreases at lower temperatures. This behaviour is indicative of weak ferromagnetic interactions coexisting with a dominant antiferromagnetic coupling. All these features have been modelled by treating this compound as a uniformly spaced antiferromagnetic linear chain with ferromagnetic interactions between the chains ( Supplementary Fig. S4 ). The bridging chloride ligand provides the magnetic pathway for the antiferromagnetic exchange ( J =−4.46 cm −1 ) and the N–H···Cl and C–H···Cl hydrogen bonds might be responsible for the weak ferromagnetic coupling ( J ′=+1.70 cm −1 ). The small value of J is consistent with the structural features. The out-of-plane bridging framework created by the packing of the square-planar Cu II units linked through the chloride ligand is not favourable to promote any exchange interaction, as the magnetic orbital of the Cu II is mainly delocalized in the equatorial plane and a very weak spin density is expected on its axial position. The different magnetic response on HCl chemisorption/desorption is confirmed by the field dependence of the magnetization measured at 2 K ( Fig. 5 ). The strong antiferromagnetic nature of coordination polymer 1 is evident due to the weak M versus H linear signal, which is much below the Brillouin function and the expected saturation value for an isolated spin S =½ ( M sat =1 μ B ). For compound 2 , the magnetization increase is sharper than that of the Brillouin function and saturates at 5 T, whereas for 3 the magnetization values are always below the Brillouin function and does not reach saturation. These results agree with the weak ferromagnetic ( 2 ) and weak antiferromagnetic ( 3 ) exchange interactions found in these compounds. EPR response to HCl chemisorption and monitoring The substantial changes in coordination environments of the copper centres due to the sorption/desorption processes permit the use of EPR spectroscopy, which is strongly sensitive to the coordination environment of the metal centres and lead to clear differences in the EPR spectra of these compounds, to monitor these structural changes. EPR spectra for 1 and 3 at different temperatures ( Supplementary Figs S2 and S5 ) show axial spectra with g || =2.25 and g ┴ = 2.08 ( g average =2.13) and g || =2.28 and g ┴ = 2.08 ( g average =2.14), respectively. These values, with g || > g ┴ , indicate a dx 2 −y 2 magnetic orbital and are in agreement with the coordination environment of the Cu. In addition, the Δ m s =±2 transition characteristic of dimeric species is not observed at the half-field region, in agreement with the dimensionality of the systems ( J -uniform magnetic chains). For 2 , EPR shows an isotropic signal at room temperature with g =2.20, which splits below 100 K ( Fig. 6 and Supplementary Fig. S6 ). The isotropic spectra observed at room temperature fully agrees with an unresolved spectra arising from the distorted tetrahedral environment exhibited by the Cu site. However, at low temperatures, an inverse axial spectrum with g || < g ┴ is found (with g || =2.100 and g ┴ = 2.255; g average =2.20), indicating a dz 2 magnetic orbital, which is unusual for distorted tetrahedral environments but typical for penta-coordinated Cu(II) complexes with trigonal bipyramid geometries [38] . This might be due to the presence of a Cu–Cl···Cu interaction ( Supplementary Fig. S7 ) that results in a pseudo-pentacoordination of the Cu atom, which is closer to a trigonal bipiramid than to a square pyramidal geometry. Hence, the anisotropy of the EPR spectra below 100 K can be seen as the result of an intermediate situation between trigonal bipyramid (from the pseudopentacoordination of the Cu) and distorted tetrahedral (from the real tetracoordination of the Cu), which implies a ground state described by a mixture of the dx 2 −y 2 and dz 2 Cu(II) orbitals and explains that g || < g ┴ . Previous studies on the variation of the EPR spectra of [CuCl 5 ] 3− with temperature [39] support this point of view. In that work, Reinen and Friebel show that the g anisotropy increases considerably on cooling down due to a change in the geometry of the [CuCl 5 ] 3− polyhedra as a consequence of a second-order Jahn–Teller effect. The situation in compound 2 is somewhat similar: at room temperature there are isolated [CuCl 4 ] 2− anions with isotropic g values; on cooling down, weak Cu–Cl···Cu interactions appear, which produce a splitting of the EPR signal. Such a structural change can be achieved owing to the high plasticity of the [CuCl 4 ] 2− anions. Nevertheless, this small g-anisotropy has no effect on the magnetic description of compound 2 ( Supplementary Fig. S8 ). 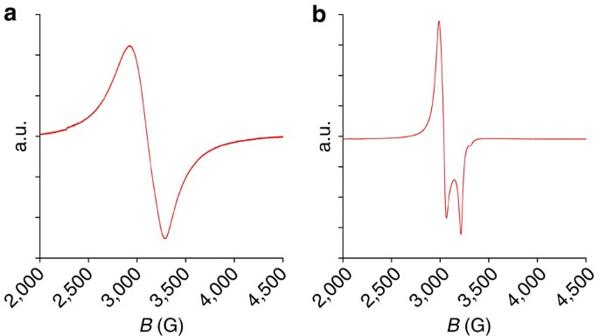Figure 6: X-band EPR spectra of compound2at different temperatures. (a) At 300 K an isotropic spectra can be observed withg=2.20, which fully agrees with an unresolved spectra that can be associated to the distorted tetrahedral environment exhibited by the Cu site. (b) At low temperatures, an inverse axial spectrum withg||<g┴is found (g||=2.100 andg┴= 2.255;gaverage=2.20), indicating a dz2magnetic orbital. This anisotropy ofgis due to a change of geometry of the Cu centre and may be caused by the presence of a Cu–Cl···Cu non-bonding interaction, which results in a pseudo-pentacoordination of the Cu, implying a ground state described by a mixture of the dx2−y2and dz2Cu(II) orbitals. Figure 6: X-band EPR spectra of compound 2 at different temperatures. ( a ) At 300 K an isotropic spectra can be observed with g =2.20, which fully agrees with an unresolved spectra that can be associated to the distorted tetrahedral environment exhibited by the Cu site. ( b ) At low temperatures, an inverse axial spectrum with g || < g ┴ is found ( g || =2.100 and g ┴ = 2.255; g average =2.20), indicating a dz 2 magnetic orbital. This anisotropy of g is due to a change of geometry of the Cu centre and may be caused by the presence of a Cu–Cl···Cu non-bonding interaction, which results in a pseudo-pentacoordination of the Cu, implying a ground state described by a mixture of the dx 2 −y 2 and dz 2 Cu(II) orbitals. Full size image The changes from the distorted tetrahedral geometry in 2 to a square-planar copper centre in 3 lead to clear differences in the room-temperature EPR spectra of these two compounds, as shown in Fig. 7a . Although both compounds present broad signals at room temperature, they are clearly distinct. More important than their difference in shape is that their resonance fields, at which their EPR signals are zero, are centred at different values (3079 G for 2 and 3209 G for 3 , see arrows in Fig. 7a ). This provides with the opportunity to monitor the position of the switch and the ratio of 2 and 3 at a given point by measuring the EPR signals at these two fields. Hence, when fixing the field at 3079 G there is no contribution of compound 2 to the EPR signal, whereas the EPR signal of 3 is very close to its maximum value. This permits the precise quantification of 3 . In addition, when fixing the field at 3209 G, the reverse situation is found: only compound 2 contributes to the EPR signal, and its value is very close to the minimum. Therefore, these two signals afford a good estimation of the composition of a mixture of 2 and 3 at room temperature ( Supplementary Fig. S9 and Supplementary Table S1 ). Interestingly, we show that the uptake/release of HCl is totally reversible and can be repetitively switched 'on' and 'off' ( Fig. 7b ), demonstrating the responsive behaviour of this magnetic molecular material. 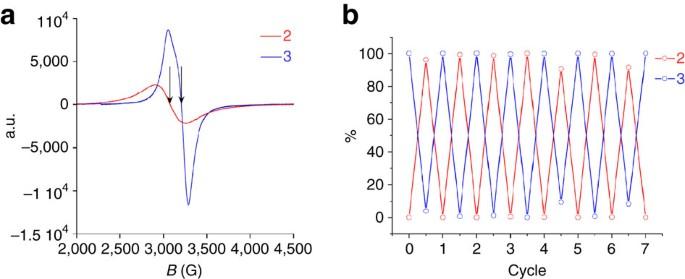Figure 7: Monitored EPR signals at room temperature. (a) X-band EPR spectra of compounds2(red) and3(blue) showing broad signals at 300 K for both compounds. Arrows indicate the resonance fields at which their EPR signals are zero, centred at different values (3079 G for2and 3209 G for3). These two signals afford a good estimation of the composition of a mixture of2and3at room temperature. (b) 'On/off' switching between crystalline2and3monitored at room temperature. The uptake–release of HCl is totally reversible and can be repetitively switched 'on' and 'off', demonstrating the responsive behaviour of this magnetic molecular material. Figure 7: Monitored EPR signals at room temperature. ( a ) X-band EPR spectra of compounds 2 (red) and 3 (blue) showing broad signals at 300 K for both compounds. Arrows indicate the resonance fields at which their EPR signals are zero, centred at different values (3079 G for 2 and 3209 G for 3 ). These two signals afford a good estimation of the composition of a mixture of 2 and 3 at room temperature. ( b ) 'On/off' switching between crystalline 2 and 3 monitored at room temperature. The uptake–release of HCl is totally reversible and can be repetitively switched 'on' and 'off', demonstrating the responsive behaviour of this magnetic molecular material. Full size image Porous coordination polymers (or MOFs) have provided many examples in which the physisorption of guest molecules provoke subtle changes in the framework that affect their magnetic properties. Here we have presented the possibility of tuning magnetic properties through gas uptake in the absence of pores. As there is no possibility of a 'guest molecule' being accommodated within pores, the gas molecules react with the material being therefore incorporated as part of the network as a result of significant chemical changes and atomic motions within the crystalline solid. Specifically, we show that chemisorption of HCl by a non-porous coordination polymer can be used as a novel approach to design responsive molecular materials with tunable magnetic properties in which gaseous HCl molecules are incorporated into the framework after cleavage of multiple covalent bonds. Crystalline [Cu(pyim)(Cl)(MeOH)] ( 1 ) displays a two-step irreversible-reversible chemisorption process, which causes substantial changes in the geometry and connectivity between the metal centres, leading to three different compounds that exhibit distinct magnetic properties. Thus, 1 forms antiferromagnetic chains of pentacoordinated square pyramidal Cu centres. On chemisorption of three equivalents of HCl molecules, the resultant ionic solid, (H 2 pyimH)[CuCl 4 ] ( 2 ), presents ferromagnetic interactions between the distorted tetrahedral [CuCl 4 ] 2− anions. Although this process is not fully reversible, compound 2 is able to extrude two equivalents of HCl yielding the molecular compound cis -[CuCl 2 (pyimH)] ( 3 ), where the square planar Cu centres show antiferromagnetic interactions. The magneto-structural switching of these materials arises from the presence of labile copper(II) centres within the coordination network, which are capable of reacting with gaseous HCl or releasing HCl in a cyclic manner without loss of effectiveness. Importantly, these non-porous frameworks display a considerable flexibility with the guest uptake and release, which do not disrupt the crystallinity of the compounds. Thus, structural analysis from single crystal diffraction and ab initio structure determination from powder diffraction has been essential to rationalize the changes in the physical properties of these compounds. In addition, we can take advantage of the switch observed in the magnetic properties on HCl chemisorption to monitor the progress of the sorption/desorption processes in these crystalline solids and, in particular, the reversible inter-conversion 2 3 . However, the magnetic changes caused by the structural transformations in these compounds are only observable in the low temperature region (below 10 K) except for compound 1 , as the magnetic susceptibility is primarily sensitive to the magnetic interactions, which are quite weak in both 2 and 3 . Interestingly, the substantial changes in coordination environments due to the sorption/desorption processes have permitted the use of EPR spectroscopy to monitor the reaction at room temperature due to its high sensitivity to the coordination environment of the metal centres. The preparation of porous magnetic materials is not easy because magnetic coupling between spin sources is often weak in the porous network. Thus, the possibility of modifying the physical properties of a material by chemisorption, despite it being non-porous, provides an important and significant step forward. At the same time, it offers an alternative route to overcoming the difficulty in combining porosity and magnetic cooperativity. This new approach for the design of chemically responsive magnetic MOFs with the absence of pores should have broad applicability across a number of areas in chemistry and materials science. Crystal syntheses and gas–solid reactions Compound 1 was synthesized in high yield as dark green needles by slow diffusion in an H-tube of methanolic solutions of CuCl 2 ·2H 2 O (34 mg, 0. 2 mmol, in 2 ml of MeOH) and 2-(imidazol-2–yl)pyridine [40] (29 mg, 0.2 mmol, in 2 ml of MeOH) in the presence of NEt 3 (28 μl, 0.2 mmol). Needle-shaped dark green single crystals of both chiralities (noted as 1+ and 1− ) were obtained after several weeks in quantitative yield in the product, which is a racemic mixture with no dichroic signal in the solid state ( Supplementary Fig. S10 ). Exposure of 30 mg (0.1 mmol) of crystalline 1 to vapours of concentrated aqueous HCl (37%) resulted in conversion to compound 2 as a microcrystalline solid and was accompanied by a colour change from dark green to yellow. The change of colour occurred within minutes, but the reaction was allowed to occur over a period of 1 day to ensure completion. A small single crystal suitable for X-ray single crystal diffraction was found among the crystalline powder. Compound 2 was left uncovered and a change in colour from yellow to bright green was observed after 1 h, resulting in conversion to compound 3 . The reaction was allowed to continue for 1 day to ensure completion. Analysis (calcd., found for C 8 H 7 N 3 Cl 2 Cu, 3 ): C (34.36, 33.79), H (2.52, 2.55), N (15.03, 15.01). No single crystals suitable for X-ray diffraction were found, and the structure was established by XRPD. Phase purity of 1–3 was checked using XRPD and EPR spectroscopy. Structural characterization Single crystals of compounds 1+ , 1– and 2 were mounted on glass fibres using a viscous hydrocarbon oil to coat the crystal and then transferred directly to the cold nitrogen stream for data collection. X-ray data were collected at 120 K on a Supernova diffractometer equipped with a graphite-monochromated Enhance (Mo) X-ray Source ( λ =0.71073 Å). The program CrysAlisPro, Oxford Diffraction Ltd., was used for unit cell determinations and data reduction. Empirical absorption correction was performed using spherical harmonics, implemented in the SCALE3 ABSPACK scaling algorithm. Crystal structures were solved and refined against all F 2 values using the SHELXTL suite of programs [41] . Non-hydrogen atoms were refined anisotropically and hydrogen atoms were placed in calculated positions that were refined using idealized geometries (riding model) and assigned fixed isotropic displacement parameters. In 1+ and 1− the coordinated methanol molecules have the CH 3 group disordered over two sites and have been modelled with 51(2):49(2) and 66.7:33.3 ratios, respectively. The single crystal of compound 2 was found to be twinned as two domains related by a rotation of 180° about the a axis [0.709(2):0.291(2)]. Crystal structure solution and refinement of the model was performed using the major component with corrected intensities for the contribution of the minor component to the overlapped reflexions. A summary of the data collection and structure refinements is provided in Supplementary Table S2 . A polycrystalline sample of 3 was lightly ground in an agate mortar and pestle and filled into a 0.7 mm borosilicate capillary. Data were collected at room temperature in the 2 θ range 0–40° on beam line I11 at Diamond Light Source, UK, using λ =0.826134 Å and a wide angle (90°) PSD detector comprising multiple Mythen-2 modules [42] , [43] . A series of six pairs of scans were conducted at room temperature, each pair related by a 0.25° detector offset to account for gaps between detector modules. The resulting 12 patterns were summed to give the final pattern for structural analysis. The diffraction pattern was indexed using DICVOL91 [44] to a monoclinic cell [F(18)=71.0, M(18)=19.8] and space group P 2 1 / n was assigned from volume considerations and a statistical consideration of the systematic absences. The data set was background subtracted and truncated to d =2.795 Å (2 θ =17.00°), for Pawley refinement [45] and the structure was solved ab initio using the simulated annealing (SA) global optimization procedure implemented in the DASH computer program [46] , [47] . The SA structure solution involved the optimization of four independent fragments in the asymmetric unit (one Cu atom, two Cl atom and one pyimH ligand), totalling 16 degrees of freedom. Z matrices describing the molecular topology of the fragments in each compound were generated automatically for all fragments using DASH. Global optimization of all external (rotational and translational) degrees of freedom against the extracted intensities was carried out with all DASH SA control parameters set to default values. 10 runs with 5×10 7 SA moves per run were implemented for structure determination. The best SA solutions had a chemically reasonable packing arrangement, and exhibited no significant misfit to the data. The solved structure was used as starting model for Rietveld refinement, conducted using TOPAS [48] . All atomic positions and displacement parameters, U iso , of non-hydrogen atoms were refined (one for Cu atom, one for all Cl atoms and one for all C and N atoms; H atoms were fixed at idealized positions and the atomic displacement parameters were set as 1.2 times those of non-hydrogen atoms), subject to a series of restraints on bond lengths, bond angles and planarity of the aromatic rings. A March–Dollase correction of the intensities for preferred orientation was applied in the final stage of refinement. Rietveld refinement [49] converged to R wp =0.02267, R ′ wp =0.07678 ( R ′ wp is the background-subtracted R wp ).The observed and calculated diffraction patterns for the refined crystal structures are shown in Fig. 4 . A summary of the data collection and structure refinements is provided in Supplementary Table S3 . Crystal data Crystal data for 1+ : trigonal, space group P 3 2 , T =120 K, a =9.6491(3) Å, b =9.6491(3) Å, c =10.7075(6) Å, V =863.36(6) Å 3 , Z =3, ρ calcd =1.588 Mg m −3 , R 1( F )=0.0699, wR 2( F 2 )=0.1647. Crystal data for 1− :trigonal, space group P 3 1 , T =120 K, a =9.6388(5) Å, b =9.6388(5) Å, c =10.6890(8) Å, V =860.03(9) Å 3 , Z=3, ρ calcd =1.594 Mg m −3 , R 1( F )=0.0651, wR 2( F 2 )=0.1166. Crystal data for 2 : monoclinic, space group Pc , T =120 K, a =6.9831(10) Å, b =7.2397(9) Å, c =12.931(2) Å, β = 105.067(15) °, V =631.28(15) Å 3 , Z =2, ρ calcd =1.855 Mg m −3 , R 1( F )=0.0546, wR 2( F 2 )=0.1506. Crystal data for 3 : monoclinic, space group P 2 1 / n , T =120 K, a =15.6450(2) Å, b =15.5700(3) Å, c =3.91545(8) Å, β =94.722(2) °, V =950.54(3) Å 3 , Z =4, ρ calcd =1.954 Mg m −3 , R wp =0.02267, R ′ wp =0.07678. Supplementary Data 1 CCDC-852548 ( 1+ ), CCDC-852549 ( 1− ), CCDC-852550 ( 2 ) and CCDC-852551 ( 3 ) contain the supplementary crystallographic data for this paper. These data can be obtained free of charge from The Cambridge Crystallographic Data Centre via http://www.ccdc.cam.ac.uk/data_request/cif . Physical measurements Magnetic susceptibility measurements were performed on single-phased polycrystalline samples with a Quantum Design SQUID magnetometer. The susceptibility data were corrected from the diamagnetic contributions as deduced by using Pascal's constant tables. The d.c. data were collected in the range 2–300 K for decreasing temperatures with an applied field of 1000 G and field dependent magnetization were collected at 2 K with an applied magnetic field increased from 0 to 5 T. EPR spectroscopy was recorded with a Bruker ELEXYS E580 spectrometer operating in the X-band (9.47 GHz). Circular dichroism of compound 1 was measured with a JASCO J-810 circular dichroism spectrometer (with a 150 W Xe lamp). How to cite this article: Coronado, E. et al . Tuning the magneto-structural properties of non-porous coordination polymers by HCl chemisorption. Nat. Commun. 3:828 doi: 10.1038/ncomms1827 (2012).